A Diels–Alder super diene breaking benzene into C2H2and C4H4units Cyclic polyene with six carbon atoms (benzene) is very stable, whereas cyclic polyene with four carbon atoms (cyclobutadiene) is extremely unstable. The electron-withdrawing pentafluorophenyl group of a substituted cyclobutadiene lowers the energy of the lowest unoccupied molecular orbital, greatly increasing its reactivity as a diene in Diels–Alder reactions with acetylene, ethylene and even benzene. Here we show that the reaction with benzene occurs cleanly at the relatively low temperature of 120 °C and results in the formal fragmentation of benzene into C 2 H 2 and C 4 H 4 units, via a unique Diels–Alder/retro-Diels–Alder reaction. This is a new example of the rare case where breaking the C–C bond of benzene is possible with no activation by a transition metal. Aromaticity is one of the fundamental concepts of organic chemistry. According to Hückel’s rule, monocyclic systems containing [4 n +2] π electrons are aromatic, while systems containing 4 n π electrons are antiaromatic [1] , [2] . Benzene, with six π electrons, has special characteristics attributed to aromaticity, such as equivalent C–C bonds, inertness towards addition reactions and so on. Cyclobutadiene, with four π electrons, is anti-aromatic and has a planar, monocyclic structure with bond alternation and high reactivity, which is attributed to its high-lying highest occupied molecular orbital (HOMO) and low-lying lowest unoccupied molecular orbital (LUMO). The archetypal example of cyclobutadiene reactivity is the Diels–Alder reaction. In fact, cyclobutadienes with small substituents are sufficiently reactive to dimerize via a Diels–Alder reaction and can also be trapped with a large variety of dienophiles [3] , [4] , [5] . Even isolable cyclobutadienes, with bulky substituents, undergo Diels–Alder cyclization with a variety of reagents [6] , [7] , [8] , [9] . However, aside from the dimerization process, cyclobutadienes almost exclusively react as electron-rich dienes. In contrast to cyclobutadiene, benzene rarely participates in Diels–Alder reactions. Only a limited number of examples of the Diels–Alder reaction involving benzene derivatives have been reported [10] , [11] , [12] , [13] , [14] , [15] , [16] , [17] . The limited reactivity of this π system is because of the enormous stability afforded by aromaticity, which can only be overcome under certain conditions [18] . Currently, there are only a limited number of options to activate benzene sufficiently, including coordination of a transition metal complex to benzene [10] , naphthalene with small resonance energy [11] and the use of benzene derivatives with a sterically induced strained geometry [12] , [13] , [14] . Alternatively, exceptionally strong dienophiles or dienes under severe conditions (for example, high temperature and pressure) will undergo Diels–Alder cyclization with benzene [15] , [16] , [17] , [18] , [19] , [20] , [21] , and reactive unsaturated heavier main group analogues of an alkene or alkyne make adducts with arenes under mild conditions [22] , [23] , [24] . As a rather peculiar case, 1,4-addition of benzene to a dihydrocyclopent[ a ]indene diradical is also reported [25] . However, the activation of benzene and its use as a diene or dienophile remain as challenges in organic chemistry. Cyclobutadienes are a valence isomer of tetrahedranes and often serve as a convenient precursor in the synthesis of these highly strained cage compounds, particularly tetrakis(trimethylsilyl)tetrahedrane. We have reported a variety of silyl-substituted tetrahedranes starting from this single precursor, including pentafluorophenyltris(trimethylsilyl)tetrahedrane ( 1 ), in recent years [26] , [27] , [28] , [29] . However, we recently reported that tetrahedranes can also be used as the precursor to synthesize new types of cyclobutadienes. In fact, tetrahedrane 1 can be efficiently photochemically isomerized into pentafluorophenyltris(trimethylsilyl)cyclobutadiene ( 2 ), which is a rare example of cyclobutadiene with two different substituents [30] . In addition, the presence of the highly electron-withdrawing pentafluorophenyl group on the cyclobutadiene ring could lead to unique Diels–Alder reactivity, such as inverse electron-demand Diels–Alder cyclization. Here to investigate this, cyclobutadiene 2 is reacted with acetylene and ethylene, two examples of unactivated dienophiles. Furthermore, during the course of our investigations we find that 2 also reacts with benzene cleanly at the relatively low temperature of 120 °C. This reaction involves the formal fragmentation of benzene into C 2 H 2 and C 4 H 4 units. Diels–Alder reactions of cyclobutadiene 2 Dried acetylene or ethylene gas was bubbled into a toluene solution of pentafluorophenyltris(trimethylsilyl)cyclobutadiene 2 for 5 min to afford Dewar benzene 3 (in 79% yield) or bicyclo[2.2.0]hex-2-ene 4 (in 82% yield), respectively ( Fig. 1 ). In both cases, the red colour of 2 disappeared within 3 min of the introduction of gas into the reaction vessel. Compounds 3 and 4 could be isolated and were fully characterized by NMR, mass spectrometry and X-ray diffraction analysis. For the molecular structures of 3 and 4 determined by X-ray crystallography, see Supplementary Figs 1 and 5 , respectively. 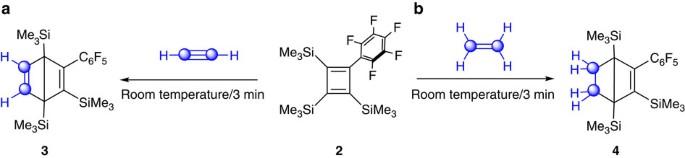Figure 1: Diels–Alder reactions of2with acetylene and ethylene. Reaction of2with (a) acetylene and (b) ethylene. Figure 1: Diels–Alder reactions of 2 with acetylene and ethylene. Reaction of 2 with ( a ) acetylene and ( b ) ethylene. Full size image We found that on heating a solution of 2 in benzene to 120 °C for 15 h in a sealed reaction tube, benzene derivative 5 , cyclooctatetraene derivative 6 and tetracyclodecadiene derivative 7 could be isolated in 25, 24 and 19% yields, respectively ( Fig. 2 ). 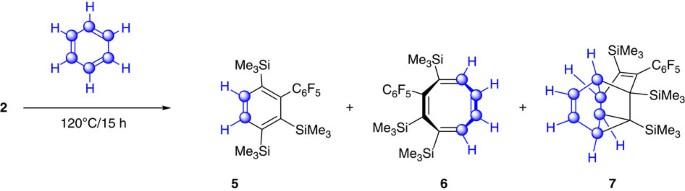Figure 2: Reaction of 2 with benzene. Products5,6and7observed in the reaction between2and benzene. Figure 2: Reaction of 2 with benzene. Products 5 , 6 and 7 observed in the reaction between 2 and benzene. Full size image The thermal reaction of 2 was also performed in benzene- d 6 . A mixture of 2 , benzene- d 6 and hexane was sealed in a reaction tube and heated at 140 °C for 14 h. After purification using HPLC, compounds 5- d 2 , 6- d 4 and 7- d 6 were obtained as colourless crystals (12%), a pale yellow oil (9%) and colourless crystals (17%), respectively. The formation of the products 5 , 6 , 7 , 5- d 2 , 6- d 4 and 7- d 6 clearly indicates that the solvent serves as a reagent in the reaction and that the C 2 H 2 unit in compound 5 and the C 4 H 4 unit in compound 6 originate from benzene, while 7 is a thermal isomerization product of the Diels–Alder cycloadduct of 2 and benzene. Compounds 5 , 6 , 7 , 5- d 2 , 6- d 4 and 7- d 6 were characterized by NMR and mass spectrometry, and the molecular structures of 5 and 7 were confirmed by X-ray diffraction analysis ( Supplementary Fig. 9 for 5 ). 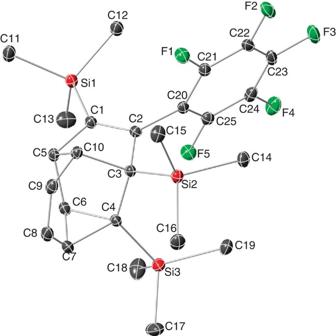Figure 3: Molecular structure of7determined by X-ray crystallography. ORTEP view of7synthesized by the reaction of the cyclobutadiene2with benzene (thermal ellipsoids are given at the 30% probability level). Hydrogen atoms are not shown. Selected bond lengths (Å): C1–C2=1.3505(16), C2–C3=1.5553(15), C1–C5=1.5303(15), C3–C4=1.5739(16), C5–C6=1.5235(16), C3–C10=1.5975(15), C5–C10=1.5566(16), C4–C6=1.5197(16), C4–C7=1.5726(16), C6–C7=1.5220(17), C7–C8=1.4616(18), C8–C9=1.3296(19), C9–C10=1.4877(16), C1–Si1=1.8756(12), C2–C20=1.4842(15), C3–Si2=1.9136(12), C4–Si3=1.8896(12). Selected bond angles (degree): C5–C1–C2=105.45(10), C1–C2–C3=110.11(10), C2–C3–C4=103.90(9), C1–C5–C6=105.86(9), C3–C4–C6=103.22(9), C5–C6–C4=105.71(9), C3–C10–C5=93.26(8), C4–C6–C7=62.26(8), C6–C7–C4=58.80(7), C7–C4–C6=58.94(8), C7–C8–C9=117.01(11), C8–C9–C10=115.45(11). Figure 3 shows the molecular structure of 7 determined by X-ray crystallography. Figure 3: Molecular structure of 7 determined by X-ray crystallography. ORTEP view of 7 synthesized by the reaction of the cyclobutadiene 2 with benzene (thermal ellipsoids are given at the 30% probability level). Hydrogen atoms are not shown. Selected bond lengths (Å): C1–C2=1.3505(16), C2–C3=1.5553(15), C1–C5=1.5303(15), C3–C4=1.5739(16), C5–C6=1.5235(16), C3–C10=1.5975(15), C5–C10=1.5566(16), C4–C6=1.5197(16), C4–C7=1.5726(16), C6–C7=1.5220(17), C7–C8=1.4616(18), C8–C9=1.3296(19), C9–C10=1.4877(16), C1–Si1=1.8756(12), C2–C20=1.4842(15), C3–Si2=1.9136(12), C4–Si3=1.8896(12). Selected bond angles (degree): C5–C1–C2=105.45(10), C1–C2–C3=110.11(10), C2–C3–C4=103.90(9), C1–C5–C6=105.86(9), C3–C4–C6=103.22(9), C5–C6–C4=105.71(9), C3–C10–C5=93.26(8), C4–C6–C7=62.26(8), C6–C7–C4=58.80(7), C7–C4–C6=58.94(8), C7–C8–C9=117.01(11), C8–C9–C10=115.45(11). Full size image The effects of concentration and temperature The effects of concentration and temperature on the ratio of the products were investigated in an effort to understand the mechanism. The concentration of 2 was varied and the ratio of the products 5 , 6 and 7 was estimated by 1 H NMR spectroscopy. Under concentrated conditions, the yields of 5 and 6 increased, while in dilute solution the yield of 7 increased ( Supplementary Fig. 19 , right). The reaction temperature was also varied and the ratio of the products 5 , 6 and 7 was estimated ( Supplementary Fig. 19 , left). At low temperature, the yields of 5 and 6 increased, while at high temperature the yield of 7 increased. In both cases, the ratio of 5 to 6 is always ~1:1. In this section, we discuss the reaction mechanism of 2 with benzene, resulting in the fragmentation of benzene into C 2 H 2 and C 4 H 4 . As mentioned above, benzene is generally very inert towards any type of cyclization reaction, and therefore cyclobutadiene 2 must have very particular electronic properties to promote this reactivity. To understand the unique nature of 2 , we set about examining the results of all of the Diels–Alder cycloaddition reactions of 2 . The reactions with acetylene and ethylene proceeded cleanly and regioselectively, and all of the cycloadditions occurred at the C–C bond substituted by two trimethylsilyl groups. From these results, a plausible mechanism for the reaction of 2 with benzene could be proposed ( Fig. 4 ). In the first step, 2 reacts in the expected role as a diene, with one double bond of the benzene taking the role of dienophile. The result of this Diels–Alder reaction is the cycloadduct A , which can subsequently isomerize at an elevated temperature to give dihydronaphthalene intermediate B . To test this possibility, the relative energies of 2 , benzene, A and B were calculated at the M06–2X/6-311+G(d,p) level. For compound 2 , two possible electronic states (closed-shell singlet and triplet) were calculated (for optimized structures, see Supplementary Fig. 21 (closed-shell singlet) and 22 (triplet)). Their relative energies are the following: 0 kcal mol −1 for the closed-shell singlet (optimized at M06–2X/6-311+G(d,p) level, see Supplementary Table 1 ) and +9.5 kcal mol −1 for the triplet (optimized at UM06-2X/6-311+G(d,p) level, see Supplementary Table 2 ), respectively. On the basis of these considerations, we discuss about only the closed-shell singlet state of 2 . For the details of the theoretical calculations on the two electronic states of 2 , see the Supplementary Methods . 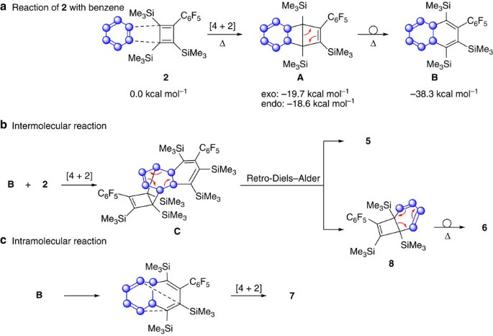Figure 4: Proposed mechanism for the thermal reaction of2with benzene. (a) The proposed mechanism for the reaction of2with benzene to form intermediateAfollowed by isomerization ofAtoB. (b) Proposed intermolecular reaction ofBwith the cyclobutadiene2, forming the products5and6through the Retro-Diels–Alder reaction ofC. (c) Proposed intramolecular reaction ofB, giving the product7. Figure 4: Proposed mechanism for the thermal reaction of 2 with benzene. ( a ) The proposed mechanism for the reaction of 2 with benzene to form intermediate A followed by isomerization of A to B . ( b ) Proposed intermolecular reaction of B with the cyclobutadiene 2 , forming the products 5 and 6 through the Retro-Diels–Alder reaction of C . ( c ) Proposed intramolecular reaction of B , giving the product 7 . Full size image The results show that the energy of intermediate A is lower than the sum of the energies of 2 and benzene (by −18.6 kcal mol −1 for endo, Supplementary Fig. 23 and Supplementary Table 3 and –19.7 kcal mol −1 for exo, Supplementary Fig. 24 and Supplementary Table 4 ). What is more interesting is that the isomerized intermediate B is, in fact, more stable than the starting materials (by −38.3 kcal mol −1 , Supplementary Fig. 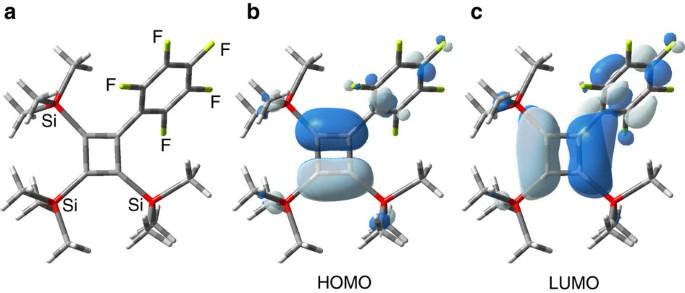Figure 5: Calculated structure of2and frontier molecular orbitals. (a) Calculated structure of2at the M06–2X/6-311+G(d,p) level. (b) Highest occupied molecular orbital (HOMO) of2. (c) Lowest unoccupied molecular orbital (LUMO) of2. 25 and Supplementary Table 5 ). This explains why isomerization becomes thermodynamically favourable once the cycloadduct A is formed. After initial formation of B , an intramolecular cycloaddition and an intermolecular cycloaddition of B with 2 compete. In the former case, B undergoes an intramolecular [4+2] cycloaddition to give compound 7 , which is one of the isolated products. In the latter case, B reacts with another equivalent of cyclobutadiene 2 ; however, in this case the C=C bond of 2 reacts as the dienophile and B reacts as the diene to give intermediate C . On a retro-Diels–Alder reaction of C , benzene 5 and bicyclo[4.2.0]octa-2,4,7-triene 8 , a valence isomer of cyclooctatetraene, are produced. Strained compound 8 subsequently thermally isomerizes to cyclooctatetraene 6 via disrotatory cleavage of the central bond in 8 (refs 31 , 32 , 33 , 34 ). This mechanism, therefore, can account for the formation of all three of the isolated products of this reaction. The effects of concentration and temperature on the ratio of the products also support the proposed mechanism. In both cases, the ratio of 5 to 6 is always approximately unity ( Supplementary Fig. 19 ), which indicates that compounds 5 and 6 could be produced from the retro-Diels–Alder reaction of C as described above. In addition, the fact that the yield of 7 , the product obtained by an intramolecular cycloaddition, increases under the dilute and high-temperature conditions ( Supplementary Fig. 19 ) agrees with the proposed mechanism. In concert, these results strongly support the mechanism described above. To gain further insight into the extraordinary reactivity of 2 , its frontier orbital energy levels were calculated at the M06−2X/6−311+G(d,p) level: the molecular orbitals of 2 (closed-shell singlet; shown in Fig. 5 ), the frontier orbital energy level of 2 and the parent cyclobutadiene C 4 H 4 (closed-shell singlet, Supplementary Fig. 26 and Supplementary Table 6 ). The HOMO level of 2 (−6.82 eV) is almost the same as that of the parent cyclobutadiene C 4 H 4 (−6.79 eV), whereas the LUMO level of 2 (−1.54 eV) is significantly lower than that of the parent cyclobutadiene (–0.79 eV; see Supplementary Fig. 20 ). Clearly, this decrease in LUMO energy can be explained by the electronic effects of the silyl and pentafluorophenyl groups; however, the strong electron-withdrawing character of the latter probably plays the most significant role in this change. This large difference between the MOs of the parent cyclobutadiene and 2 clearly indicates that this unprecedented reactivity of 2 towards benzene is caused by the low-energy LUMO. Next, the frontier orbital levels of acetylene, ethylene and benzene were also calculated at the M06−2X/6−311+G(d,p) level ( Supplementary Figs 27–29 , Supplementary Tables 7–9 ), and the energy differences between the frontier orbitals of 2 and these dienophiles were compared. The LUMO levels of benzene (0.45 eV), ethylene (0.75 eV) and acetylene (0.71 eV) are very similar, while HOMO levels are decreased in the order of benzene (−8.42 eV), ethylene (−9.14 eV) and acetylene (−9.75). In the case of benzene, LUMO diene /HOMO dienophile interactions are favoured over the HOMO diene /LUMO dienophile interactions (for the energy levels of the frontier orbitals, see Supplementary Fig. 20 ), while in the case of ethylene and acetylene the interaction is reversed because of their low-lying HOMOs (HOMO diene /LUMO dienophile interactions are favoured over the LUMO diene /HOMO dienophile interactions). That is, the electron-withdrawing pentafluorophenyl substituent would make 2 an electron-poor diene and, consequently, 2 would participate in inverse electron-demand Diels–Alder reactions towards benzene. Figure 5: Calculated structure of 2 and frontier molecular orbitals. ( a ) Calculated structure of 2 at the M06–2X/6-311+G(d,p) level. ( b ) Highest occupied molecular orbital (HOMO) of 2 . ( c ) Lowest unoccupied molecular orbital (LUMO) of 2 . Full size image In summary, cyclobutadiene 2 , with an electron-withdrawing pentafluorophenyl group, has an extremely low-lying LUMO, which facilitates Diels–Alder reactions with the unreactive benzene. The role of benzene as a dienophile or a diene in Diels–Alder reaction is determined depending on the reacting partner. In the majority of the reported Diels–Alder reactions involving benzene (for example, with benzynes) benzene reacts as a diene, while in our case benzene reacts as a dienophile. In the reaction of 2 with benzene, formal fragmentation of the benzene ring into C 2 H 2 and C 4 H 4 units is involved. Mechanistically, a retro-Diels–Alder reaction is the key step in this fragmentation. This is a rare case of benzene participating in a cycloaddition reaction without activation by transition metals or the use of extreme conditions. Synthesis of bicyclo[2.2.0]hexa-2,5-diene 3 A toluene solution of pentafluorophenyltris(trimethylsilyl)cyclobutadiene 2 (100 mg, 0.230 mmol) was prepared, and dried acetylene gas was bubbled into the solution for 5 min. On bubbling, the red colour of the solution disappeared within 3 min. The solvent was removed under vacuum and the residue was purified using HPLC (eluent t BuOMe:MeOH=1:1). Compound 3 was obtained as colourless crystals (83.2 mg, 79%); melting point (mp): 83–86 °C; 1 H NMR (400 MHz, C 6 D 6 ): δ –0.03 (s, 9H, Si Me 3 ), −0.02 (s, 9H, SiMe 3 ), 0.18 (s, 9H, SiMe 3 ), 6.56 (d, 1H, 3 J (HH)=2.3 Hz, CH), 6.76 (dd, 1H, 3 J (HH)=2.3 Hz, J (HF)=3.0 Hz, CH); 13 C NMR (101 MHz, C 6 D 6 ): δ −1.7 (SiMe 3 ), −1.1 (SiMe 3 ), −0.4 (SiMe 3 ), 63.7 ( C -SiMe 3 ), 65.0 ( C -SiMe 3 ), 114.0 (t, 2 J (CF)=19 Hz, ipso - C 6 F 4 ), 137.6 (d, 1 J (CF)=255 Hz, C 6 F 4 ), 137.8 (d, 1 J (CF)=259 Hz, C 6 F 4 ), 140.6 (d, 1 J (CF)=254 Hz, C 6 F 4 ), 142.2 (d, J (CF)=3 Hz, CH), 143.1 (d, J (CF)=5 Hz, CH), 145.3 (d, 1 J (CF)=253 Hz, C 6 F 4 ), 145.8 (d, 1 J (CF)=234 Hz, C 6 F 4 ), 151.0 (C-C 6 F 4 ), 162.8 (C-SiMe 3 ); 29 Si NMR (79 MHz, C 6 D 6 ): δ –11.5, –3.8, –3.1; high-resolution mass spectrometry (HRMS) (atmospheric pressure chemical ionization (APCI)) ( m / z ): [M] + calcd. for C 21 H 29 F 5 Si 3 , 460.1492; found, 460.1484. For copies of 1 H, 13 C and 29 Si NMR spectra see Supplementary Figs 2–4 . Crystal data for 3 at 120 K: molecular formula (MF)=C 21 H 29 F 5 Si 3 , molecular weight (MW)=460.71 daltons, orthorhombic, space group Pbca , a =11.6307(5) Å, b =12.5277(5) Å, c =33.4761(14) Å, V =4877.7(4) Å 3 , Z =8, D calcd =1.255 g cm −3 . The final R factor was 0.0426 ( R w =0.1254 for all data) for 25,785 reflections with I >2 σ ( I ), goodness-of-fit (GOF)=1.025. Synthesis of bicyclo[2.2.0]hexa-2-ene 4 A toluene solution of pentafluorophenyltris(trimethylsilyl)cyclobutadiene 2 (100 mg, 0.230 mmol) was prepared, and dried ethylene gas was bubbled into this solution for 5 min. On bubbling, the red colour of the solution disappeared within 3 min. The solvent was removed under vacuum and the residue was purified using HPLC (eluent t BuOMe:MeOH=1:1). Compound 4 was obtained as colourless crystals (87.0 mg, 82%); mp 75–78 °C; 1 H NMR (400 MHz, C 6 D 6 ): δ −0.10 (s, 9 H, SiMe 3 ), 0.01 (s, 9 H, SiMe 3 ), 0.12 (s, 9H, SiMe 3 ), 1.69–1.75 (m, 1H, CH 2 ), 2.15–2.27 (m, 3H, CH 2 ); 13 C NMR (101 MHz, C 6 D 6 ): δ −2.0 (SiMe 3 ), −1.3 (SiMe 3 ), −0.9 (SiMe 3 ), 23.6 (CH 2 ), 23.7 (CH 2 ), 53.1 (C-SiMe 3 ), 55.3 (C-SiMe 3 ), 114.4 (t, 2 J (CF)=25 Hz, ipso - C 6 F 4 ), 137.8 (d, 1 J (CF)=249 Hz, C 6 F 4 ), 137.9 (d, 1 J (CF)=249 Hz, C 6 F 4 ), 140.6 (d, 1 J (CF)=254 Hz, C 6 F 4 ), 144.0 (d, 1 J (CF)=245 Hz, C 6 F 4 ), 144.6 (d, 1 J (CF)=249 Hz, C 6 F 4 ), 150.0 (C-C 6 F 4 ), 164.4 (C-SiMe 3 ); 29 Si NMR (79 MHz, C 6 D 6 ): δ −13.7, −3.1, −2.7; HRMS (APCI) ( m / z ): [M] + calcd. for C 21 H 31 F 5 Si 3 , 462.1648; found, 462.1647. For copies of 1 H, 13 C and 29 Si NMR spectra see Supplementary Figs 6–8 . Crystal data for 4 at 120 K: MF=C 21 H 31 F 5 Si 3 , MW=462.73, orthorhombic, space group Pbca , a =11.6585(7) Å, b =12.5084(7) Å, c =33.328(2) Å, V =4860.1(5) Å 3 , Z=8, D calcd =1.265 g cm −3 . The final R factor was 0.0334 ( R w =0.0937 for all data) for 25,372 reflections with I >2 σ ( I ), GOF=1.040. Reaction of cyclobutadiene 2 with benzene A benzene solution (14 ml) of pentafluorophenyltris(trimethylsilyl)cyclobutadiene 2 (140 mg, 0.322 mmol) was sealed in a reaction tube. The solution of 2 was heated at 120 °C for 15 h. The colour of the solution gradually changed from red to pale yellow on heating. The solvent was removed under vacuum and the reaction mixture was purified using HPLC (eluent t BuOMe:MeOH=1:1). Compounds 5 , 6 and 7 were obtained as colourless crystals (36.8 mg, 25%), a pale yellow oil (37.4 mg, 24%) and colourless crystals (30.9 mg, 19%), respectively. The corresponding deuterated compounds 5- d 2 , 6- d 4 and 7- d 6 were obtained by a similar procedure in hexane (12 ml) and benzene- d 6 (2 ml). The solution of 2 (97.7 mg, 0.225 mmol) was heated at 140 °C for 14 h. After purification using HPLC (eluent t BuOMe:MeOH=1:1), compounds 5- d 2 , 6- d 4 and 7- d 6 were obtained as colourless crystals (12.2 mg, 12%), a pale yellow oil (9.7 mg, 9%) and colourless crystals (19.3 mg, 17%), respectively. Spectral and crystallographic data for 5 Compound 5 : mp 95–97 °C; 1 H NMR (400 MHz, C 6 D 6 ): δ −0.06 (s, 9 H, SiMe 3 ), 0.04 (s, 9H, SiMe 3 ), 0.33 (s, 9H, SiMe 3 ), 7.53 (d, 1H, 3 J (HH)=7.6 Hz, CH), 7.63 (d, 1H, 3 J (HH)=7.6 Hz, CH); 13 C NMR (101 MHz, C 6 D 6 ): δ −0.3 (SiMe 3 ), 3.3 (SiMe 3 ), 3.4 (SiMe 3 ), 120.3 (t, 2 J (CF)=20 Hz, ipso -C 6 F 4 ), 134.7 (CH), 136.5 (CH), 136.9 (C-C 6 F 4 ), 138.3 (d, 1 J (CF)=253 Hz, C 6 F 4 ), 140.8 ( C -SiMe 3 ), 141.3 (d, 1 J (CF)=255 Hz, C 6 F 4 ), 145.9 (d, 1 J (CF)=244 Hz, C 6 F 4 ), 147.0 (C-SiMe 3 ), 149.8 (C-SiMe 3 ); 29 Si NMR (79 MHz, C 6 D 6 ): δ −5.0, −3.8, −2.3; HRMS (APCI) ( m / z ): [M] + calcd. for C 21 H 29 F 5 Si 3 , 460.1492; found, 460.1517. For copies of 1 H, 13 C and 29 Si NMR spectra see Supplementary Figs 10–12 . Crystal data for 5 at 120 K: MF=C 21 H 29 F 5 Si 3 , MW=460.71, orthorhombic, space group Pca2(1) , a =19.1914(10) Å, b =10.6017(5) Å, c =23.3513(12) Å, V =4,751.1(4) Å 3 , Z=8, D calcd =1.288 g cm −3 , The final R factor was 0.0282 ( R w =0.0664 for all data) for 25,588 reflections with I >2 σ ( I ), GOF=0.989. Spectral data for 6 1 H NMR (400 MHz, C 6 D 6 ): δ −0.11 (s, 9 H, SiMe 3 ), −0.07 (s, 9 H, SiMe 3 ), 0.21 (s, 9 H, SiMe 3 ), 5.89 (dd, 1 H, 3 J (HH)=11.6 Hz, 3 J (HH)=3.3 Hz, CH), 5.91 (d, 1H, 3 J (HH)=2.8 Hz, CH), 6.04 (dd, 1H, 3 J (HH)=11.6 Hz, 3 J (HH)=2.8 Hz, CH), 6.08 (d, 1H, 3 J (HH)=3.3 Hz, CH); 13 C NMR (101 MHz, C 6 D 6 ): δ –0.5 (SiMe 3 ), 0.5 (d, J (CF)=3 Hz, SiMe 3 ), 1.1 (SiMe 3 ), 118.0 (t, 2 J (CF)=22 Hz, ipso -C 6 F 4 ), 131.8 (CH), 133.4 (CH), 134.9 (C-C 6 F 4 ), 135.8 (CH), 138.1 (d, 1 J (CF)=252 Hz, C 6 F 4 ), 138.3 (d, 1 J (CF)=252 Hz, C 6 F 4 ), 141.0 (d, 1 J (CF)=254 Hz, C 6 F 4 ), 141.8 (CH), 144.5 (d, 1 J (CF)=243 Hz, C 6 F 4 ), 145.9 (d, 1 J (CF)=250 Hz, C 6 F 4 ), 148.7 (C-SiMe 3 ), 155.1 (C-SiMe 3 ), 155.5 (C-SiMe 3 ); 29 Si NMR (79 MHz, C 6 D 6 ): δ −7.9, −5.9, −4.3; HRMS (APCI) ( m / z ): [M] + calcd. for C 23 H 31 F 5 Si 3 , 486.1648; found, 486.1675. For copies of 1 H, 13 C and 29 Si NMR spectra see Supplementary Figs 13–15 . Spectral and crystallographic data for 7 Compound 7 : mp 97–101 °C; 1 H NMR (400 MHz, CDCl 3 ): δ −0.14 (d, 9H, J (HF)=1.3 Hz, SiMe 3 ), −0.09 (s, 9H, SiMe 3 ), 0.03 (d, 9H, J (HF)=1.8 Hz, SiMe 3 ), 1.69 (ddd, 1H, 3 J (HH)=6.6 Hz, 3 J (HH)=1.5 Hz, 4 J (HH)=1.0 Hz, CH), 2.10 (dd, 1H, 3 J (HH)=1.5 Hz, 5 J (HH)=1.5 Hz, CH), 2.53 (ddd, 1H, 3 J (HH)=6.6 Hz, 3 J (HH)=6.3 Hz, 4 J (HH)=2.0 Hz, CH), 2.58 (dd, 1H, 3 J (HH)=7.1 Hz, 4 J (HH)=1.0 Hz, CH), 5.98 (ddd, 1H, 3 J (HH)=8.3 Hz, 3 J (HH)=7.1 Hz, 4 J (HH)=2.0 Hz, CH), 6.51 (ddd, 1H, 3 J (HH)=8.3 Hz, 3 J (HH)=6.3 Hz, 5 J (HH)=1.5 Hz, CH); 13 C NMR (101 MHz, CDCl 3 ): δ −1.3 (SiMe 3 ), 1.1 (d, J (CF)=2 Hz, SiMe 3 ), 1.4 (d, J (CF)=4 Hz, SiMe 3 ), 29.7 (C-SiMe 3 ), 37.7 (CH), 38.3 (CH), 49.2 (CH), 52.8 (C-SiMe 3 ), 61.1 (CH), 116.9 (t, 2 J (CF)=21 Hz, ipso -C 6 F 4 ), 127.7 (CH), 129.2 (CH), 137.4 (d, 1 J (CF)=252 Hz, C 6 F 4 ), 137.6 (d, 1 J (CF)=251 Hz, C 6 F 4 ), 140.3 (d, 1 J (CF)=254 Hz, C 6 F 4 ), 143.3 (d, 1 J (CF)=239 Hz, C 6 F 4 ), 144.9 (d, 1 J (CF)=246 Hz, C 6 F 4 ), 150.8 (C-C 6 F 4 ), 162.3 (C-SiMe 3 ); 29 Si NMR (79 MHz, CDCl 3 ): δ –8.9, –0.9, 3.8; HRMS (APCI) ( m / z ): [M] + calcd. for C 25 H 33 F 5 Si 3 , 512.1805; found, 512.1805. For copies of 1 H, 13 C and 29 Si NMR spectra see Supplementary Figs 16–18 . Crystal data for 7 at 120 K: MF=C 25 H 33 F 5 Si 3 , MW=512.78, triclinic, space group P-1 , a =9.6564(3) Å, b =11.3871(4) Å, c =12.9349(4) Å, α =72.10°, β =81.25°, γ =79.77°, V =1324.69(7) Å 3 , Z =2, D calcd =1.286 g cm −3 . The final R factor was 0.0294 ( R w =0.0804 for all data) for 15,018 reflections with I >2 σ ( I ), GOF=1.038. Theoretical calculations The details of the theoretical calculations are provided in the Supplementary Methods . Accession codes: Details the structure of 3 , 4 , 5 and 7 have been deposited with the Cambridge Crystallographic Data Centre under the Accession code 921572 – 921575 , respectively, and are available free of charge at www.ccdc.cam.ac.uk/data_request/cif . How to cite this article: Inagaki, Y. et al. A Diels–Alder super diene breaking benzene into C 2 H 2 and C 4 H 4 units. Nat. Commun. 5:3018 doi: 10.1038/ncomms4018 (2014).